ProteinL-isoaspartyl methyltransferase regulates p53 activity Protein methylation plays important roles in most, if not all, cellular processes. Lysine and arginine methyltransferases are known to regulate the function of histones and non-histone proteins through the methylation of specific sites. However, the role of the carboxyl-methyltransferase protein L -isoaspartyl methyltransferase (PIMT) in the regulation of protein functions is relatively less understood. Here we show that PIMT negatively regulates the tumour suppressor protein p53 by reducing p53 protein levels, thereby suppressing the p53-mediated transcription of target genes. In addition, PIMT depletion upregulates the proapoptotic and checkpoint activation functions of p53. Moreover, PIMT destabilizes p53 by enhancing the p53–HDM2 interaction. These PIMT effects on p53 stability and activity are attributed to the PIMT-mediated methylation of p53 at isoaspartate residues 29 and 30. Our study provides new insight into the molecular mechanisms by which PIMT suppresses the p53 activity through carboxyl methylation, and suggests a therapeutic target for cancers. Protein l-isoaspartyl methyltransferase (PIMT), the 'protein repair enzyme', specifically methylates the isoaspartyl residue generated by the spontaneous deamidation of asparagine, and this methylation is an essential step for converting isoaspartate to aspartate [1] . Because asparagine deamidation, which is primarily found in aged proteins, impairs protein function [2] , [3] , most studies of PIMT focus on elucidating its role in protein repair [1] , [4] . However, recent studies have shown that asparagine deamidation regulates normal cellular processes, including synaptic transmission [5] , cellular matrix interactions [6] , [7] , [8] , [9] , lifespan [10] , [11] and apoptosis [12] , [13] , [14] , [15] . Thus, the PIMT-mediated methylation of isoaspartate may also be involved in normal biological processes. Research to date has suggested that PIMT is linked to apoptosis, which is an essential cellular process for cell death. These studies show that the induction of PIMT protects cells from apoptosis caused by H 2 O 2 stress [16] or Bax overexpression [17] , whereas the inhibition of PIMT increases apoptosis upon DNA damage [18] . In addition, the effect of PIMT on apoptosis is mediated through modulating the deamidation of Bcl-xL [16] , [19] . Although these results raise the possibility that PIMT could be a regulator of apoptosis, the precise molecular mechanisms of PIMT in apoptosis have yet to be defined. p53 is a potent tumour suppressor and regulates several cellular processes, including metabolic homeostasis, DNA repair, growth arrest, senescence and apoptosis. p53 is involved in various signal pathways by interacting with cellular proteins, and its activity is regulated by different post-translational modifications, such as ubiquitination, phosphorylation, acetylation, ribosylation and glycosylation [20] . Recently, it was also found that the activity and cellular functions of p53 are regulated by lysine or arginine methylation of specific site in p53 [21] , [22] , [23] , [24] , [25] , [26] . However, the role of carboxyl methylation in p53 regulation is still unrevealed. Here we show that PIMT suppresses the activity of p53 through destabilizing p53 by enhancing the p53–HDM2 interaction, which leads to the inhibition of p53 target gene expression. We also find that PIMT methylates p53 at isoaspartate residues 29 and 30, which is required to negatively regulate the p53 activity. Collectively, we suggest carboxyl methylation as a post-translational modification of p53, providing an alternative function of PIMT in p53 regulation. PIMT is associated with the p53 pathway To examine the clinical relevance of PIMT, we dichotomized lung ( n =442) and breast ( n =404) cancer patients according to the expression levels of PIMT using publicly available gene expression data [27] , [28] , [29] . The survival of patients exhibiting higher expression of PIMT levels was significantly poorer than those with lower expression levels ( Fig. 1a ). These data suggest that the increased expression of PIMT might be a key genetic event during cancer development. On the basis of these findings and previous observations [16] , [17] , [18] , [19] , we hypothesized that PIMT could be involved in regulating the function of p53, which is a potent tumour suppressor and major regulator of apoptosis. To test this hypothesis, we examined the expression levels of PIMT and p53 in several cell lines. The level of p53 protein was generally anti-parallel with that of PIMT protein, particularly in the NTERA2 and NCCIT cells derived from poorly differentiated aggressive tumours ( Fig. 1b ). To gain insight into the influence of PIMT on the p53 pathway, we tested the effect of PIMT depletion using short interfering RNA (siRNA) and short hairpin RNA (shRNA), and found that reduction in the levels of PIMT increased the p53 protein levels in U2OS cell ( Fig. 1c,d ). The effects of PIMT depletion on the level of endogenous p53 protein were confirmed in other cancer cell lines ( Fig. 1e ). Conversely, the ectopic expression of PIMT decreased the p53 protein levels in a dose-dependent manner ( Fig. 1f ). In addition, the expression of PIMT in the PIMT-depleted cells suppressed the increase of p53 protein levels, suggesting that the effect of PIMT is specific ( Fig. 1g ). PIMT knockdown in U2OS cells did not affect the MEK and AKT signalling pathways that regulate the p53 protein levels ( Supplementary Fig. S1a–c ). Overall, these data demonstrate that PIMT negatively regulates p53 protein levels. 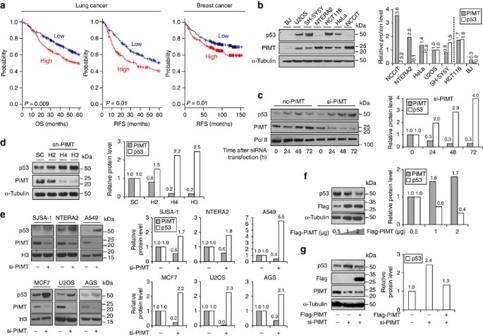Figure 1: PIMT regulates p53 protein levels. (a) A significant association of PIMT expression in human lung (n=442) and breast cancer (n=404) was found with the overall survival (OS) or recurrence-free survival (RFS). The data are represented as the mean±s.e.m. (b) Immunoblot analysis of cell lysates from seven different cell lines (BJ: foreskin fibroblast; U2OS: osteosarcoma; SH-SY5Y: neuroblastoma; NTERA2: embryonal carcinoma; HCT116: colorectal carcinoma; HeLa: cervical adenocarcinoma; NCCIT: embryonal carcinoma). (c) Immunoblot analysis of cell lysates from U2OS cells transfected with PIMT siRNA or control siRNA for the indicated times. (d) Immunoblot analysis of cell lysates from U2OS cells transfected with three different PIMT shRNA constructs (H2, H3 and H4) or scramble shRNA (SC). (e) Immunoblot analysis of cell lysates from several cancer cell lines transfected with PIMT siRNA or control siRNA. (f) Immunoblot analysis of cell lysates from U2OS cells transfected with the indicated amounts of the Flag-PIMT expression vector. (g) Immunoblot analysis of cell lysates from U2OS cells transfected with PIMT siRNA targeting a non-CDS sequence of the PIMT mRNA (line 2), followed by transfection with the Flag-PIMT expression vector (line 3). The relative protein levels were measured by Image Gauge software (version 3.12) and described as histograms to the right of each blot. Figure 1: PIMT regulates p53 protein levels. ( a ) A significant association of PIMT expression in human lung ( n =442) and breast cancer ( n =404) was found with the overall survival (OS) or recurrence-free survival (RFS). The data are represented as the mean±s.e.m. ( b ) Immunoblot analysis of cell lysates from seven different cell lines (BJ: foreskin fibroblast; U2OS: osteosarcoma; SH-SY5Y: neuroblastoma; NTERA2: embryonal carcinoma; HCT116: colorectal carcinoma; HeLa: cervical adenocarcinoma; NCCIT: embryonal carcinoma). ( c ) Immunoblot analysis of cell lysates from U2OS cells transfected with PIMT siRNA or control siRNA for the indicated times. ( d ) Immunoblot analysis of cell lysates from U2OS cells transfected with three different PIMT shRNA constructs (H2, H3 and H4) or scramble shRNA (SC). ( e ) Immunoblot analysis of cell lysates from several cancer cell lines transfected with PIMT siRNA or control siRNA. ( f ) Immunoblot analysis of cell lysates from U2OS cells transfected with the indicated amounts of the Flag-PIMT expression vector. ( g ) Immunoblot analysis of cell lysates from U2OS cells transfected with PIMT siRNA targeting a non-CDS sequence of the PIMT mRNA (line 2), followed by transfection with the Flag-PIMT expression vector (line 3). The relative protein levels were measured by Image Gauge software (version 3.12) and described as histograms to the right of each blot. Full size image PIMT inhibits the activity of p53 To investigate the effects of PIMT on p53 function further, we examined whether PIMT regulates p53 target gene expression. Among the genes activated by p53, the depletion of PIMT resulted in the expression of p21 , HDM2 , PUMA and TSP1 ( Fig. 2a,b ), whereas PIMT knockdown reduced the expression of CD44 , a gene that is normally repressed by p53 ( Fig. 2b ). However, upon the ectopic expression of PIMT, the expression levels of the p53 target genes were inversely proportional to those resulting from PIMT depletion ( Supplementary Fig. S2a,b ). These data indicate that PIMT represses the expression of p53 target genes. We then used H1299 cells, which lack endogenous p53, to examine whether the effect of PIMT on the target gene expression depended on p53. In the absence of p53, PIMT did not affect the expression of the p53 target genes, whereas PIMT negatively effected the expression of the p53 target genes in the H1299 cells transfected with p53 ( Supplementary Fig. S3a,b ). Moreover, the upregulation of p21 expression upon PIMT knockdown was eliminated by the co-knockdown of p53 ( Fig. 2c and Supplementary Fig. S3c ). These results indicate that PIMT represses the expression of the p53 target genes in a p53-dependent manner. 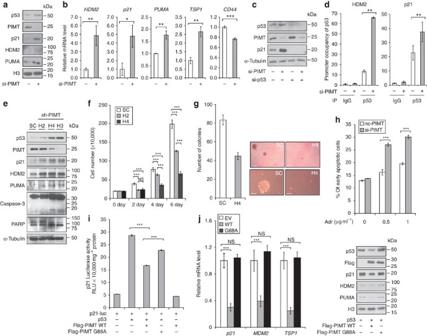Figure 2: PIMT inhibits the activity of p53. (a) Immunoblot analysis of cell lysates from U2OS cells transfected with PIMT siRNA or control siRNA. (b) Quantitative real-time PCR was used to measure the relative mRNA levels ofHDM2,p21,PUMA,TSP1andCD44in U2OS cells transfected with control siRNA or PIMT siRNA. The data are represented as the mean±s.d.,n=3. (c) Immunoblot analysis of cell lysates from U2OS cells transfected with PIMT siRNA, p53 siRNA or both. (d) Chromatin immunoprecipitation assay to assess the recruitment of p53 to the promoters of the p53-responsive element of thep21orHDM2gene in U2OS cells transfected with control siRNA or PIMT siRNA. The data are represented as the mean±s.d.,n=3. (e) Immunoblot analysis of PIMT knockdown or control stable U2OS cell lines. (f) The growth rate of the PIMT knockdown or control stable U2OS cell lines. The data are represented as the mean±s.d.,n=4. (g) Soft agar colony-forming assay using the PIMT knockdown or control stable MCF7 cell lines. The colonies were counted and visualized using nitroblue tetrazolium (NBT) staining. The data are represented as the mean±s.d.,n=3. Scale bar, 250 μM (upper panel) or 100 μM (lower panel). (h) Flow cytometry analysis of U2OS cells transfected with PIMT siRNA or control siRNA, followed by adriamycin treatment. The data are represented as the mean±s.d.,n=4. (i) Luciferase assay of cell lysates from H1299 cells transfected with expression vectors for either wild-type PIMT (WT) or mutant-type PIMT (G88A), together with p21-luc, as indicated. The data are represented as the mean±s.d.,n=4. (j) Quantitative real-time PCR or immunoblot analysis of cell lysates from U2OS cells transfected with expression vectors for either wild-type PIMT (WT) or mutant-type PIMT (G88A), as indicated. Statistical significance was analyzed using the Student'st-test and expressed as aP-value. *P<0.05; **P<0.01; ***P<0.005; NS, not significant. Figure 2: PIMT inhibits the activity of p53. ( a ) Immunoblot analysis of cell lysates from U2OS cells transfected with PIMT siRNA or control siRNA. ( b ) Quantitative real-time PCR was used to measure the relative mRNA levels of HDM2 , p21 , PUMA , TSP1 and CD44 in U2OS cells transfected with control siRNA or PIMT siRNA. The data are represented as the mean±s.d., n =3. ( c ) Immunoblot analysis of cell lysates from U2OS cells transfected with PIMT siRNA, p53 siRNA or both. ( d ) Chromatin immunoprecipitation assay to assess the recruitment of p53 to the promoters of the p53-responsive element of the p21 or HDM2 gene in U2OS cells transfected with control siRNA or PIMT siRNA. The data are represented as the mean±s.d., n =3. ( e ) Immunoblot analysis of PIMT knockdown or control stable U2OS cell lines. ( f ) The growth rate of the PIMT knockdown or control stable U2OS cell lines. The data are represented as the mean±s.d., n =4. ( g ) Soft agar colony-forming assay using the PIMT knockdown or control stable MCF7 cell lines. The colonies were counted and visualized using nitroblue tetrazolium (NBT) staining. The data are represented as the mean±s.d., n =3. Scale bar, 250 μM (upper panel) or 100 μM (lower panel). ( h ) Flow cytometry analysis of U2OS cells transfected with PIMT siRNA or control siRNA, followed by adriamycin treatment. The data are represented as the mean±s.d., n =4. ( i ) Luciferase assay of cell lysates from H1299 cells transfected with expression vectors for either wild-type PIMT (WT) or mutant-type PIMT (G88A), together with p21-luc, as indicated. The data are represented as the mean±s.d., n =4. ( j ) Quantitative real-time PCR or immunoblot analysis of cell lysates from U2OS cells transfected with expression vectors for either wild-type PIMT (WT) or mutant-type PIMT (G88A), as indicated. Statistical significance was analyzed using the Student's t -test and expressed as a P -value. * P <0.05; ** P <0.01; *** P <0.005; NS, not significant. Full size image The effects of PIMT on p53 target gene expression suggested that PIMT might regulate p53-dependent transcriptional activity. Thus, we used a luciferase construct linked to a p21 or Bax promoter, which are well-characterized p53 target genes, to address this possibility and found that PIMT inhibited the p53-dependent transcription of both reporter genes ( Supplementary Fig. S4a,b ). Using a chromatin immunoprecipitation assay, we investigated whether PIMT could affect the p53 occupancy at the promoters of its target genes and observed that PIMT depletion induced p53 occupancy at the p21 and HDM2 promoters ( Fig. 2d ). These data indicate that PIMT negatively affects the transcriptional activity of p53. Because PIMT reduced p53 target gene expression and repressed the transcriptional activity of p53, we speculated that PIMT might inhibit the cellular functions of p53. To determine whether PIMT could suppress the response of p53 to DNA damage, we measured the expression of p53 target genes upon DNA damage. Under genotoxic stress, PIMT depletion induced the expression of p53 target genes, including p21 , HDM2 , TSP1 , 14-3-3 , PUMA and GADD45 ( Supplementary Fig. S5a–c ); however, the expression of CD44 and BIRC5 , genes that are normally repressed by p53, was reduced by PIMT depletion ( Supplementary Fig. S5c ). In contrast, the expression of the p53 target genes was suppressed by the ectopic expression of PIMT ( Supplementary Fig. S6a,b ). These data indicate that PIMT inhibits p53 target gene expression upon DNA damage. We next addressed the role of PIMT in apoptosis and cell-cycle arrest. Using lentivirus-mediated PIMT shRNA, we generated three stable cell lines with different PIMT expression patterns that contrasted with the p53 expression patterns. Consistent with the induction of p53 in these cells, the expression of the p53 target genes was also upregulated. Furthermore, the active caspase-3 and poly-(ADP-ribose) polymerase cleavage levels, which are well-known apoptosis markers, were increased in the PIMT knockdown stable cell lines ( Fig. 2e ). Compared with the control, the growth rate of the PIMT knockdown stable cell lines was reduced and correlated with the reduction of PIMT expression ( Fig. 2f and Supplementary Fig. S7a ). In addition, the PIMT knockdown stable cell lines displayed a lower efficiency of colony formation in soft agar, a phenotype that is representative of cell transformation ( Fig. 2g ). Upon DNA damage, the PIMT knockdown rendered the cells more prone to apoptosis compared with the control cells (30.1% early apoptosis in the PIMT-depleted cells versus 19.5% for the control cells treated with 1 μg ml −1 adriamycin) ( Fig. 2h ). These data were also confirmed in the PIMT knockdown stable cell lines ( Supplementary Fig. S7b ). These results suggest that PIMT represses apoptosis and growth arrest through the negative regulation of the p53 activity. The methylase activity of PIMT is required to regulate p53 We then sought to determine whether the methylase activity of PIMT was required for modulating the p53 activity. To this end, we mutated glycine 88 (G88) within motif I, a residue that is critical for the methylase activity of PIMT [30] , [31] . The overexpression of this PIMT mutant, if not all, failed to reduce the p53 transactivation activity and p53 target gene expression ( Fig. 2i,j ). These data were also confirmed in H1299 cells through the ectopic expression of p53 ( Supplementary Fig. S8a,b ). These results demonstrate that the methylase activity of PIMT is necessary for regulating p53 activity. PIMT interacts with p53 To clarify the role of PIMT in p53 regulation, we confirmed that PIMT could interact with p53. p53 was found to co-immunoprecipitate with PIMT in H1299 cells co-expressing PIMT and p53 ( Fig. 3a,b ). Using MCF7 or U2OS cells, the reciprocal immunoprecipitation with PIMT demonstrated the interaction with endogenous p53, and this interaction was disrupted by adriamycin treatment ( Fig. 3c,d ). These data indicate that PIMT interacts with p53. 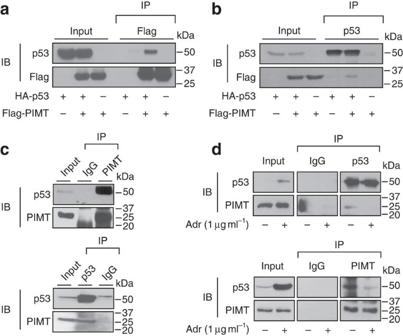Figure 3: PIMT interacts with p53. (a) Immunoblot analysis of Flag immunoprecipitates (IP line) and cell lysates (Input line) from H1299 cells transfected with the expression vector for Flag-PIMT and HA-p53. (b) Immunoblot analysis of p53 immunoprecipitates (IP line) and cell lysates (Input line) from H1299 cells transfected with the expression vector for Flag-PIMT and HA-p53. (c) Immunoblot analysis of PIMT immunoprecipitates (upper panel) and p53 immunoprecipitates (lower panel) from MCF7 cells. (d) Immunoblot analysis of p53 immunoprecipitates (upper panel) and PIMT immunoprecipitates (lower panel) from U2OS cells treated with adriamycin. Figure 3: PIMT interacts with p53. ( a ) Immunoblot analysis of Flag immunoprecipitates (IP line) and cell lysates (Input line) from H1299 cells transfected with the expression vector for Flag-PIMT and HA-p53. ( b ) Immunoblot analysis of p53 immunoprecipitates (IP line) and cell lysates (Input line) from H1299 cells transfected with the expression vector for Flag-PIMT and HA-p53. ( c ) Immunoblot analysis of PIMT immunoprecipitates (upper panel) and p53 immunoprecipitates (lower panel) from MCF7 cells. ( d ) Immunoblot analysis of p53 immunoprecipitates (upper panel) and PIMT immunoprecipitates (lower panel) from U2OS cells treated with adriamycin. Full size image PIMT methylates asparagine residues 29 and 30 of p53 Because PIMT interacted with p53 and its methylase activity was necessary for regulating p53, we examined whether PIMT directly methylates p53. Using an in vitro methylation assay, we found that PIMT methylated p53, whereas the PIMT G88A mutant did not ( Fig. 4a and Supplementary Fig. S9a ). To determine the specific region of p53 methylation, we performed the in vitro methylation assay using truncated p53. The N terminus of p53 (amino acids 1–82) was methylated by PIMT, but not by the PIMT G88A mutant ( Fig. 4b,c ). Moreover, these methylations were removed upon alkaline treatment, confirming that the p53 methylations were specifically attributed to carboxyl methylation and not lysine or arginine methylation ( Fig. 4d ). We then generated several mutants in which selected asparagine or aspartate residues were replaced with alanine residues, and then performed in vitro methylation assays. The substitution of N29 or N30 with alanine (N29A or N30A) in the N terminal of p53 mostly abolished the PIMT-mediated methylation ( Fig. 4e ). To confirm that PIMT methylates p53 at isoaspartate residues 29 and 30, we synthesized peptides consisting of amino acids 22–40 of p53, in which asparagines 29 and 30 were replaced with isoaspartates (N29IsoD, N30IsoD and N29,30IsoD). Using in vitro methylation assay, we found that PIMT methylated N29IsoD, N30IsoD and N29,30IsoD, but not the wild-type p53 peptide ( Fig. 4f and Supplementary Fig. S9b ). We also observed a 14 Da mass shift for both N29IsoD and N30IsoD, but not for the p53 peptide containing asparagine residues 29 and 30 ( Supplementary Fig. S9c ). Furthermore, we identified 14 and 28 Da mass shifts for the p53 peptide, N29,30IsoD ( Supplementary Fig. S9c ). In consistent with this result, the substitution of N29 and N30 with alanine in the full-length p53 (N29,30A) resulted in the depletion of the PIMT-mediated methylation ( Fig. 4g ). Nano-flow liquid chromatography-coupled electro spray ionization tandem mass spectrometry (nano-LC-ESI-MS/MS) analysis also confirmed the methylations at IsoD29 and IsoD30 in the recombinant p53 ( Supplementary Fig. S9d ). These data indicate that asparagine 29 and 30 could be target sites for PIMT-mediated p53 methylation. 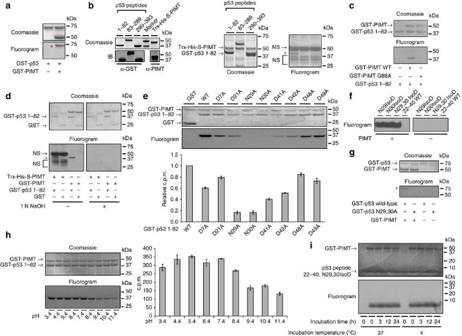Figure 4: PIMT methylates p53 at N29 and N30. (a) Fluorography results of the methylation assay using recombinant GST-PIMT on GST-p53. Asterisk indicates methylated GST-p53. (b) Immunoblot (IB) analysis of purified recombinant GST-PIMT and GST-p53 peptides 1–82, 83–289 and 290–393 (left panel). Fluorography results of the methylation assay using recombinant GST-PIMT and GST-p53 peptides 1–82, 83–289 or 290–393 (right panel). NS means nonspecific. Asterisk indicates methylated GST-p53 (1–82). (c) Fluorography results of the methylation assay using recombinant GST-PIMT (wild-type) or GST-PIMT (G88A) and GST-p53 peptides 1–82. (d) Fluorography results of the methylation assay using recombinant GST-PIMT or His-PIMT and GST-p53 peptides 1–82, followed by NaOH treatment, as indicated. NS means nonspecific. Asterisk indicates methylated GST-p53 (1–82). (e) Fluorography results of the methylation assay using recombinant GST-PIMT and GST-p53 peptides 1–82 or GST-p53 peptides 1–82 bearing D7A, D21A, N29A, N30A, D41A, D42A, D48A or D49A replacements (upper panel). A liquid scintillation counter (LSC) was used to measure the relative c.p.m. (counts per minute) of each sample (lower panel). The data are represented as the mean±range,n=2. (f) Fluorography of the methylation assay with recombinant GST-PIMT and p53 peptides, as indicated. (g) Fluorography of the methylation assay with recombinant GST-PIMT and the full-length p53 mutant (N29,30A). Asterisks indicate methylated GST-p53 wild-type. Asterisk indicates methylated GST-p53. (h) Fluorography of methylated GST-p53 peptide incubated in Tris buffer under several pH conditions. LSC was used to measure the relative c.p.m. of each sample. The data are represented as the mean±range,n=2. (i) Fluorography of the methylated p53 peptides incubated for different time intervals at 37 °C or 4 °C in Tris buffer. Figure 4: PIMT methylates p53 at N29 and N30. ( a ) Fluorography results of the methylation assay using recombinant GST-PIMT on GST-p53. Asterisk indicates methylated GST-p53. ( b ) Immunoblot (IB) analysis of purified recombinant GST-PIMT and GST-p53 peptides 1–82, 83–289 and 290–393 (left panel). Fluorography results of the methylation assay using recombinant GST-PIMT and GST-p53 peptides 1–82, 83–289 or 290–393 (right panel). NS means nonspecific. Asterisk indicates methylated GST-p53 (1–82). ( c ) Fluorography results of the methylation assay using recombinant GST-PIMT (wild-type) or GST-PIMT (G88A) and GST-p53 peptides 1–82. ( d ) Fluorography results of the methylation assay using recombinant GST-PIMT or His-PIMT and GST-p53 peptides 1–82, followed by NaOH treatment, as indicated. NS means nonspecific. Asterisk indicates methylated GST-p53 (1–82). ( e ) Fluorography results of the methylation assay using recombinant GST-PIMT and GST-p53 peptides 1–82 or GST-p53 peptides 1–82 bearing D7A, D21A, N29A, N30A, D41A, D42A, D48A or D49A replacements (upper panel). A liquid scintillation counter (LSC) was used to measure the relative c.p.m. (counts per minute) of each sample (lower panel). The data are represented as the mean±range, n =2. ( f ) Fluorography of the methylation assay with recombinant GST-PIMT and p53 peptides, as indicated. ( g ) Fluorography of the methylation assay with recombinant GST-PIMT and the full-length p53 mutant (N29,30A). Asterisks indicate methylated GST-p53 wild-type. Asterisk indicates methylated GST-p53. ( h ) Fluorography of methylated GST-p53 peptide incubated in Tris buffer under several pH conditions. LSC was used to measure the relative c.p.m. of each sample. The data are represented as the mean±range, n =2. ( i ) Fluorography of the methylated p53 peptides incubated for different time intervals at 37 °C or 4 °C in Tris buffer. Full size image To test the stability of p53 methylation, we performed an in vitro methylation assay with purified GST-p53 and GST-PIMT, and incubated the methylated GST-p53 at 37 °C under different pH conditions. The methylation of p53 was stable at pH 6.4–8.4, a physiological pH range of cells ( Fig. 4h ). We also found that methylation of p53 peptide was maintained after incubation at 37 °C for 24 h ( Fig. 4i ). PIMT only methylates isoaspartate, which is generated by the deamidation of asparagine residue. For this reason, we next determined whether or how fast asparagine residues 29 and 30 in the p53 peptide (amino acids 22–40) are deamidated ( Fig. 5a ). PIMT methylated the p53 peptide during a 30-min incubation period and the level of methylated peptide increased with increasing incubation time ( Fig. 5b ). Nano-LC-ESI-MS/MS analysis also identified the deamidation of asparagine residues 29 and 30 in incubated p53 peptides, indicating that asparagine residues 29 and 30 of p53 can be rapidly deamidated in vitro ( Fig. 5c and Supplementary Fig. S10a–c ). 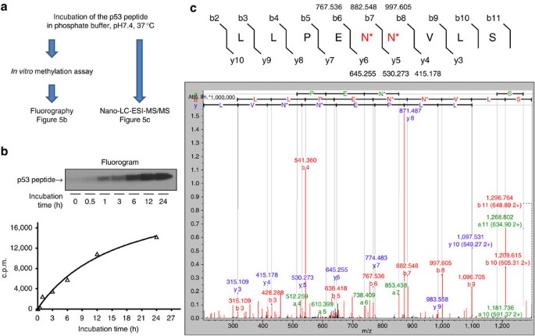Figure 5: Deamidation of p53 at N29 and N30. (a) Schematic outline of the experiment. (b) Fluorography of the methylation assay with recombinant GST-PIMT and p53 peptides 22–40 (upper panel). Liquid scintillation counting (LSC) was used to measure the c.p.m. (counts per minute) of each sample (lower panel). The data are represented as the mean±range,n=2. (c) Nano-LC-ESI-MS/MS analysis of the p53 peptide incubated for 1 h in Tris buffer. CID mode is used for MS/MS. Ion score is 65 and charge value of selected parent peptide is +2. Figure 5: Deamidation of p53 at N29 and N30. ( a ) Schematic outline of the experiment. ( b ) Fluorography of the methylation assay with recombinant GST-PIMT and p53 peptides 22–40 (upper panel). Liquid scintillation counting (LSC) was used to measure the c.p.m. (counts per minute) of each sample (lower panel). The data are represented as the mean±range, n =2. ( c ) Nano-LC-ESI-MS/MS analysis of the p53 peptide incubated for 1 h in Tris buffer. CID mode is used for MS/MS. Ion score is 65 and charge value of selected parent peptide is +2. Full size image Next, we determined whether PIMT methylates p53 under physiological conditions through nano-LC-ESI-MS/MS analysis of endogenous p53 purified from U2OS cells or ectopic-expressed p53 purified from H1299 cells under conditions in which the PIMT-catalyzed methylation of the isoaspartyl residues was stable enough for detection ( Fig. 4h,i ). We found that two asparagine residues, N29 and N30, were deamidated and methylated ( Supplementary Fig. S11a–c ); however, methyl+deamidated p53 was not detected in the PIMT knockdown U2OS cells ( Supplementary Fig. S11d ). These results confirm the PIMT-mediated methylation of endogenous p53. In addition, there are two theoretical deamidation-susceptible sites in p53, asparagine residues 239 and 268. Although we found that only one site, asparagine 268, in the endogenous p53 immunoprecipitated from the U2OS cell extracts was deamidated, we could not detect the methylation of the deamidated asparagine 268 ( Supplementary Fig. S12 ). Thus, the methylation of deamidated asparagine residues 29 and 30, but not 268, might play an important role in the regulation of p53 activity. Our sequence alignment analysis confirms that asparagine residues 29 and 30 are conserved in the nine upper vertebrate p53 proteins listed in GenBank ( Supplementary Fig. S13a ). Interestingly, the p53 proteins in Rattus norvegicus and Mus musculus do not contain conserved asparagine 29 and 30 residues. Moreover, the PIMT knockdown in three different mouse cell lines does not affect the level of p53 protein ( Supplementary Fig. S13b ). PIMT influences the stability of p53 The N29 and N30 residues are located near the domain implicated in the regulation of HDM2 binding and p53 stability ( Fig. 6a ). Furthermore, PIMT depletion upregulated the p53 protein levels without increasing the p53 mRNA levels ( Fig. 6b ). These results suggest that PIMT regulates p53 levels by destabilizing the p53 protein. To test this possibility, we investigated the effects of PIMT on the major regulation mechanism for p53 stability, degradation and ubiquitination. PIMT depletion restrained p53 degradation (half-life of p53, 58.1 min in the PIMT-depleted cells versus 8.7 min in the control cells) and reduced the ubiquitination of p53 ( Fig. 6c–e ). Conversely, the ectopic expression of PIMT increased p53 ubiquitination ( Fig. 6f ). These results suggest that PIMT positively regulates the ubiquitination and destabilization of p53. 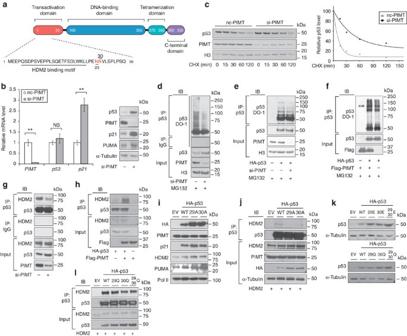Figure 6: PIMT influences the stability of p53. (a) Locations of the methylated asparagine residues in p53. (b) Immunoblot (IB) analysis and quantitative real-time PCR of cell lysates from U2OS cells transfected with control siRNA or PIMT siRNA. The data are represented as the mean±s.e.m.,n=3. (c) IB analysis of cell lysates from U2OS cells transfected with PIMT siRNA or control siRNA, followed by treatment with cycloheximide (CHX, 20 μg ml−1) for the indicated times. The relative protein levels of p53 were measured using the ImageGauge software and analyzed with GraphPad Prism 5. (d) IB analysis of p53 immunoprecipitation (IP) in U2OS cells transfected with control or PIMT siRNA, followed by treatment with MG132 (40 μM). (e) IB analysis of p53 IP in H1299 cells transfected with the expression vector for HA-p53 and PIMT siRNA, followed by MG132 treatment (40 μM). (f) IB analysis of the p53 IP in H1299 cells transfected with the expression vector for Flag-PIMT and HA-p53, followed by MG132 treatment (40 μM). (g) IB analysis of p53 IP in U2OS cells transfected with control or PIMT siRNA. (h) IB analysis of p53 IP in H1299 cells transfected with expression vectors for HA-p53 or Flag-PIMT, as indicated. (i) IB analysis of cell lysates from H1299 cells transfected with expression vectors for wild-type HA-p53 (WT) or mutant HA-p53 (N29A, N30A). (j) IB analysis of HA IP (IP panel) and cell lysates (Input panel) in H1299 cells transfected with expression vectors for either HA-p53 (WT) or mutant HA-p53 (N29A or N30A) together with HDM2, as indicated. (k) IB analysis of cell lysates from H1299 cells transfected with expression vectors for wild-type HA-p53 (WT) or mutant HA-p53 (N29E, N30E, N29,30E, N29Q, N30Q, N29,30Q). (l) IB analysis of HA IP (IP panel) and cell lysates (Input panel) in H1299 cells transfected with the expression vectors for either HA-p53 (WT) or mutant HA-p53 (N29Q, N30Q or N29,30Q) together with HDM2, as indicated. Statistical significance was analyzed using the Student'st-test and expressed as aP-value. **P<0.01; NS, not significant. Figure 6: PIMT influences the stability of p53. ( a ) Locations of the methylated asparagine residues in p53. ( b ) Immunoblot (IB) analysis and quantitative real-time PCR of cell lysates from U2OS cells transfected with control siRNA or PIMT siRNA. The data are represented as the mean±s.e.m., n =3. ( c ) IB analysis of cell lysates from U2OS cells transfected with PIMT siRNA or control siRNA, followed by treatment with cycloheximide (CHX, 20 μg ml −1 ) for the indicated times. The relative protein levels of p53 were measured using the ImageGauge software and analyzed with GraphPad Prism 5. ( d ) IB analysis of p53 immunoprecipitation (IP) in U2OS cells transfected with control or PIMT siRNA, followed by treatment with MG132 (40 μM). ( e ) IB analysis of p53 IP in H1299 cells transfected with the expression vector for HA-p53 and PIMT siRNA, followed by MG132 treatment (40 μM). ( f ) IB analysis of the p53 IP in H1299 cells transfected with the expression vector for Flag-PIMT and HA-p53, followed by MG132 treatment (40 μM). ( g ) IB analysis of p53 IP in U2OS cells transfected with control or PIMT siRNA. ( h ) IB analysis of p53 IP in H1299 cells transfected with expression vectors for HA-p53 or Flag-PIMT, as indicated. ( i ) IB analysis of cell lysates from H1299 cells transfected with expression vectors for wild-type HA-p53 (WT) or mutant HA-p53 (N29A, N30A). ( j ) IB analysis of HA IP (IP panel) and cell lysates (Input panel) in H1299 cells transfected with expression vectors for either HA-p53 (WT) or mutant HA-p53 (N29A or N30A) together with HDM2, as indicated. ( k ) IB analysis of cell lysates from H1299 cells transfected with expression vectors for wild-type HA-p53 (WT) or mutant HA-p53 (N29E, N30E, N29,30E, N29Q, N30Q, N29,30Q). ( l ) IB analysis of HA IP (IP panel) and cell lysates (Input panel) in H1299 cells transfected with the expression vectors for either HA-p53 (WT) or mutant HA-p53 (N29Q, N30Q or N29,30Q) together with HDM2, as indicated. Statistical significance was analyzed using the Student's t -test and expressed as a P -value. ** P <0.01; NS, not significant. Full size image To investigate how these effects converged on p53 ubiquitination, we next determined whether PIMT affects the interaction of HDM2 and p53 and found that the interaction was impaired by PIMT depletion and enhanced by the ectopic expression of PIMT ( Fig. 6g,h ). In addition, the binding of the p53 mutants (N29A, N30A) to HDM2 was diminished and was accompanied with an increase in the p53 protein levels ( Fig. 6i,j ). These data were also confirmed using other p53 mutants in which glutamate (E) or glutamine (Q) residues were substituted for the asparagine residues ( Fig. 6k,l ). These results indicate that methylation at N29 and N30 are necessary for the destabilization of p53, most likely through ubiquitination by enhancing the interaction of p53 and HDM2. Because deamidation of asparagine residues resulted in structural change of protein, it could affect the binding affinity of target proteins [5] , [32] . To test this, we performed surface plasmon resonance analysis using the N29,30IsoD peptide and revealed that N29,30IsoD peptide had a lower ( K D= 694 μM) HDM2 binding affinity than wild-type peptide ( K D =141 μM) ( Supplementary Fig. S14a–c ). In addition, a competitive binding assay of N29,30IsoD and methylated N29,30IsoD peptides with HDM2 showed that the methylated N29,30IsoD peptide had a higher HDM2 binding affinity than the N29,30IsoD peptide ( Supplementary Fig. S15a,b ). PIMT is a well-known carboxyl-methyltransferase that specifically methylates isoaspartyl residues. Although the enzymatic mechanism of PIMT is well established, the biological function of PIMT is controversial and far from being completely understood. Here, we reveal the critical roles of PIMT in p53 regulation. We show that PIMT suppresses p53 protein levels and target gene expression by reducing the transcriptional activity of p53. We also find that PIMT disrupts the response of p53 to DNA damage. Under genotoxic stress, PIMT inhibits the expression of damage-induced p53 target genes and protects cancer cells from apoptosis, which is the most important function of p53 in tumour suppression. Moreover, cell proliferation is impaired in the PIMT knockdown stable cell lines, as indicated by the increased p53 protein levels and target gene expression. We also demonstrate that the reduced survival rates of cancer patients are related to the increased expression of PIMT. We observe that PIMT expression is increased in several cancer cell lines, including the NTERA2 and NCCIT cells, derived from poorly differentiated aggressive tumours. Thus, we speculate that PIMT plays an important role in obstructing the tumour suppression function of p53 by modulating its activity; thus, PIMT is a potential oncogene. On the basis of our results, PIMT deserves further investigation to understand its full potential in cancer development and progression. In this study, we also reveal that p53 protein is a novel substrate for PIMT. We show that asparagine residues 29 and 30 of p53 are methylated by PIMT in vivo and in vitro . We demonstrate that PIMT depletion hinders the interaction between p53 and HDM2, resulting in an augmentation of the p53 protein. We also observe that the protein levels of p53 mutants in which asparagine residues 29 and 30 are replaced with glutamines or alanines are increased, as indicated by the reduction of their binding to HDM2. These results suggest that PIMT and its methylation of p53 are required for p53 destabilization through the enhancement of the interaction between HDM2 and p53. Because the PIMT-mediated methylation of p53 could directly regulate the interaction between HDM2 and p53, PIMT might act as a regulator for the maintenance of p53 steady-state levels, and the interaction of p53 and HDM2 could be regulated through the PIMT-mediated methylation of isoaspartyl residues. The surface plasmon resonance analysis and a competitive binding assay demonstrate that p53 deamidation impairs the binding to HDM2, while methylation of deamidated p53 enhances it ( Supplementary Figs S14a–c and S15a,b ). These observations support the hypothesis that PIMT might act as a regulator for the maintenance of p53 steady-state levels by tagging p53 for degradation rather than by repairing the isoaspartyl residues to aspartates. Although asparagine deamidation is a non-enzymatic and spontaneous reaction, it is now clear that the rate of asparagine deamidation primarily depends on the amino-acid residues near the asparagine in the peptide chain and the three-dimensional structure of the protein [33] , [34] , [35] . Several studies suggest that asparagine deamidation is not unregulated, but is genetically programmed and acts as an embedded clock that functions during the lifetime of a protein [36] , [37] . Thus, asparagine residues 29 and 30 of p53 might not be suitable for deamidation reaction because Asn–Asn–Val is an unusual deamidation-susceptible sequence [36] . However, we demonstrate that asparagine residues 29 and 30 in the p53 peptide could be rapidly deamidated in vitro , despite their unusual deamidation-susceptible sequence ( Fig. 5b,c ). Consistent with these observations, we also observe the deamidation of asparagine residues 29 and 30 in immunoprecipitated p53 in vivo ( Supplementary Fig. S11a–d ). Several studies demonstrate that the deamidation rate could also be regulated through signal-transduction pathways: the deamidation of Bcl-xL occurs in response to DNA damage [12] , [13] , [14] , [15] , [16] , [19] and is suppressed by the Rb protein [12] , the p56 lck kinase [14] , the BCR-ABL and mutant JAK2 proteins [15] . Thus, we speculate that there is a specific regulation mechanism for accelerating the asparagine deamidation of p53 in the intracellular environment, even though asparagine residues 29 and 30 of short-lived p53 are present in an unusual deamidation-susceptible sequence. Our studies are the first to elucidate the function of PIMT in p53 regulation and to uncover p53 as a novel substrate of PIMT. These results provide a previously unrecognized link between the p53 pathway and carboxyl methylation, and show that PIMT is a key regulator of the p53 pathway. We anticipate that our results will improve the current understanding of how carboxyl methylation regulates cellular processes. Plasmid construction The DNA constructs were a generous gifts from Dr Danny Reinberg [21] (pCDNA-HA-p53, pGEX-GST-p53, pGEX-GST-p53 (1–82), pGEX-GST (83–289), pGEX (290–393) and pET-His-p53) and Dr Ber Vogelstein [38] (full-length human p21 promoter luciferase). The constructs for wild-type PIMT were generated using PCR and cloned into the backbone of pCMV (Clontech), pGEX (Clontech) and pET32 (Invitrogen). The mutant constructs for p53 and PIMT were generated using site-direct mutagenesis (p53 N7A, D21A, N29A, N30A, D41A, D42A, D48A, D49A, N29 30A, N29D, N30D, N29 30D, N29E, N30E, N29 30E, N29Q, N30Q and N29,30Q, as well as PIMT G88A). All of the constructs were confirmed via sequencing. Antibodies The anti-p53 clone DO-1 (Santa Cruz Biotechnology; SC-126, SC-126AC, SC-126HRP), anti-PIMT (SC-100977, SC-133894, 1:1,000 dilution), anti-PUMA (SC-28226, 1:250 dilution), anti-HDM2 (SC-965, SC-965HRP, SC-965AC, SC-812, 1:500 dilution), anti-Bax (SC-493, 1:1,000 dilution), anti-p21 (SC-756, 1:500 dilution), anti-tubulin (SC-32293, 1:2,000 dilution), anti-Flag (Santa Cruz Biotechnology, SC-807AC; Sigma, F-3165; Abcam, ab49763HRP) and anti-HA (SC-7392HRP, 1:4,000 dilution) antibodies were used in this study. Generation of stable cell lines The lentiviral shRNA set for PIMT (shRNA H3, 5′-GCGCTAGAACTTCTATTTGAT-3′; shRNA H2, 5′-CCAGGCGCTAATAGATCAGTT-3′; and shRNA H4, 5′-GATCACATTAAAGAGCTAGTA-3′) was purchased from Open Biosystems. The lentivirus was obtained from 293TF cells according to the manufacturer's protocol. The U2OS cells were seeded onto 100 mm plates and infected with lentivirus containing the shRNA for PIMT. Cells expressing PIMT shRNA were selected using puromycin (2 μg ml −1 ). Luciferase assay H1299 cells were plated at 1×10 5 cells per well in 12-well plates and transiently transfected using Lipofectamine 2000 (Invitrogen). The total amount of plasmid DNA added to each well was adjusted to 1 μg by adding the necessary amount of empty vector. After transfection, the luciferase activities of the cell lysates were measured according to the manufacturer's instructions (Promega). The relative luciferase activity was normalized to the protein content of the cell extract [39] . Flow cytometry analysis U2OS cells were transfected with PIMT siRNA or control siRNA. At 2 days after transfection, the U2OS cells were treated with adriamycin at the indicated dose, and one day after treatment, the apoptotic cells were determined using flow cytometry. The fluorescence-activated cell sorting (FACS) analysis was performed using a FACS Canto II machine (BD Biosciences). For each treatment, a minimum of 10,000 cells was analysed. The data analysis was conducted using the DB FACSDiva software. Raw data of FACS analysis are described in Supplementary Fig. S16 . Immunoblotting and immunoprecipitation For immunoblotting, each sample was subjected to electrophoresis on 4–12% NuPAGE Bis–Tris gradient gels (Invitrogen), and the proteins were transferred to polyvinylidene difluoride membranes using semi-dry transfer (Bio-Rad). The membranes were incubated overnight with the indicated primary antibodies, followed by incubation for 1 h with the secondary antibody, which was conjugated to horseradish peroxidase (Abcam). The signals were detected using chemiluminescence reagents (Intron). For immunoprecipitation, the cells were harvested and lysed in IP lysis buffer (40 mM HEPES (pH 7.4), 120 mM NaCl, 1 mM EDTA, 50 mM NaF, 1.5 mM Na 3 VO 4 , 10 mM β-glycerophosphate, 0.30% CHAPSO and protease inhibitors) [40] . The lysates were centrifuged for 20 min at 10,000 g at 4 °C. The specific antibodies conjugated to agarose (for FLAG, HA and p53, purchased from Santa Cruz Biotechnology) were added to the supernatants for overnight incubation at 4 °C. Subsequently, the beads were pelleted for 1 min at 7,000 r.p.m. and washed two times with IP lysis buffer. The proteins were eluted in 2× Laemmli buffer (Bio-Rad) or 4× LDS sample buffer (Invitrogen) by boiling for 5 min. The immunoprecipitated proteins were subjected to immunoblotting using horseradish peroxidase-conjugated primary antibodies. Raw data of the important protein blot are described in Supplementary Fig. S16 . Protein purification Escherichia coli BL21 harbouring pGEX-GST-p53, pGEX-GST-PIMT, pET-His-p53 or pET-His-PIMT was cultured overnight at 37 °C in the LB medium containing ampicillin. Approximately 1 ml of seed culture was inoculated into 100 ml LB and cultured at 37 °C. When the culture reached OD 600, isopropyl- b - D -thiogalactopyranoside was added to 0.2–1 mM and incubated at 30 °C for 4 h. The cell pellet was lysed using a sonicator fixed with a 2-mm probe for 3 min in lysis buffer (50 mM NaH 2 PO 4 (pH 8.0), 300 mM NaCl, 1 mM dithiothreitol, 0.1 mM phenylmethyl sulphonyl fluoride and 10 μg ml −1 aprotinin) and centrifuged at 8,000 g for 20 min. A 50% Ni 2+ -NTA or glutathione S -transferase bead slurry was added to the supernatant and incubated at 4 °C for 1 h. The beads were washed three times with wash buffer. After centrifugation, the proteins were eluted with elution buffer for 30 min at 4 °C. In vitro methylation assay Purified p53 protein or p53 peptides were used for the in vitro methylation assays. Each protein was incubated in citrate-phosphate buffer (0.25 M citric acid, 0.5 M Na 2 HPO 4 , 0.02 M EDTA (pH 6.0), and 7.19 pM S -adenosyl- L -[methyl- 3 H]methionine (specific activity of 76.4 Ci mmol −1 )) at 30 °C for 30 min. The reaction was terminated upon the addition of sample buffer and subjected to electrophoresis on 4–12% NuPAGE Bis–Tris gradient gels (Invitrogen) using MES running buffer. The gels were stained with Coomassie blue R-150 to visualize the protein bands and then subjected to fluorography for 72 h at −70 °C using sensitized AGFA 100 NIF film (Agfa) or analyzed using a liquid scintillation counter (GE Healthcare). Nano-LC-ESI-(CID/ETD)-MS/MS For the p53 protein identification, trypsin, chymotrypsin or endoproteinase Asp-N peptides were separated using a biocompatible Ultimate 3000 nano-LC system (Dionex) equipped with a PepMap100 C-18 trap column (300 μm i.d.×5-mm-long cartridge, from Dionex) and PepMap100 C-18 analytic column (75 μm i.d.×150-mm-long cartridge, from Dionex). The gradient consisted of (A) 0.1% formic acid in water and (B) 0.08% formic acid in ACN: 4–30% B from 0 to 105 min, 80% B from 105 to 110 min and 4% B from 110 to 125 min. The flow rate was 300 nl min −1 from 0 to 12 min, 75 nl min −1 from 12 to 105 min and 300 nl min −1 from 105 to 125 min. An HCT ultra-PTM discovery system (Bruker Daltonics) was used to record the peptide spectra over the mass range of m / z 350–1,500 and the MS/MS spectra using information-dependent data acquisition over the mass range of m / z 100–2,800. Repeatedly, the MS spectra were recorded, followed by four data-dependent collision-induced dissociation MS/MS spectra and four electron transfer dissociations. The MS/MS spectra were generated from the four highest intensity precursor ions using the following parameters: an absolute threshold limit of 30,000 and a 25% relative threshold. The voltage between the ion spray tip and spray shield was set to 1,550 V. The drying nitrogen gas was heated to 170 °C, and the flow rate was 10 l min −1 . The collision energy was set automatically according to the mass and charge state of the peptides chosen for fragmentation. Two 3-charged peptides were chosen for the MS/MS experiments because of their good fragmentation characteristics. The MS/MS spectra were interpreted, and the peak lists were generated using DataAnalysis 4.0 (Bruker Daltonics), with the parameters set to an absolute threshold limit of 5,000 and a 0.1% relative threshold. The searches were performed using MASCOT v2.2 (Matrix Science) against the UniProtKB/Swiss-prot database (version 57.14) for protein identification. The following MASCOT searching parameters were set: enzyme selected as trypsin or Asp-N, with three maximum missing cleavage sites; species limited to human; a mass tolerance of 0.2 Da for peptide tolerance; 0.2 Da for MS/MS tolerance; ion score cutoffs lower than 20; fixed modification of carbamidomethyl (C) and variable modification of oxidation (M), deamidation (N, Q), methylation (D, E) and methyl+deamidation (N). The positive protein identifications were based on significant molecular weight search scores. After the protein identification, an error-tolerant search with set parameters was performed to detect unspecific cleavages, amino-acid substitutions and unassigned modifications [41] . Quantitative real-time PCR Total RNA was isolated using Easy-Blue (Intron). The reverse transcriptase PCR was performed using the Access RT–PCR system (Promega). The quantitative real-time PCR was performed using the KAPA™ SYBR FAST qPCR Kit (Kapabiosystems) and a CFX96™ or Chromo4™ real-time PCR detector (Bio-Rad). The relative mRNA levels were normalized to the values of GAPDH mRNA for each reaction. The primer sequences are listed in Supplementary Table S1 . Chromatin immunoprecipitation assay The chromatin immunoprecipitation assay was performed according to the manufacturer's protocol (Upstate Biotechnology). A small portion of the crosslinked, sheared chromatin solution was saved as the input DNA, and the remainder was employed for the immunoprecipitation using a p53 antibody conjugated to agarose (Santa Cruz Biotechnology). The immunoprecipitated DNAs were purified by phenol–chloroform extraction and ethanol precipitation; the DNA was re-suspended in 20 μl TE buffer. The immunoprecipitated and input DNA were analyzed using quantitative real-time PCR. Statistical analysis Statistical significance was analyzed using the Student's t -test and expressed as a P -value. How to cite this article: Lee, J.C. et al . Protein L -isoaspartyl methyltransferase regulates p53 activity. Nat. Comm. 3:927 doi: 10.1038/ncomms1933 (2012).